Turnover of soil bacterial diversity driven by wide-scale environmental heterogeneity Spatial scaling and determinism of the wide-scale distribution of macroorganism diversity has been largely demonstrated over a century. For microorganisms, and especially for soil bacteria, this fundamental question requires more thorough investigation, as little information has been reported to date. Here by applying the taxa–area relationship to the largest spatially explicit soil sampling available in France (2,085 soils, area covered ~5.3 × 10 5 km 2 ) and developing an innovative evaluation of the habitat–area relationship, we show that the turnover rate of bacterial diversity in soils on a wide scale is highly significant and strongly correlated with the turnover rate of soil habitat. As the diversity of micro- and macroorganisms appears to be driven by similar processes (dispersal and selection), maintaining diverse and spatially structured habitats is essential for soil biological patrimony and the resulting ecosystem services. Since the first statement of microbial biogeography developed by Baas Becking [1] in 1934 “Everything is everywhere, but, the environment selects”, it is now well established that soil microbial communities exhibit biogeographical patterns, that is, variations in their distribution across space and time [2] . Although the increasing number of studies of spatial microbial ecology from local to wide scale [3] is helping to identify ecological processes (selection, dispersal, ecological and evolutionary drifts, speciation) impacting microbial diversity, the hierarchy of these processes remains unclear in comparison with that of macroorganisms. One way to tackle the spatial processing of microbial diversification is to evaluate the empirical relationship between geographical distance and genetic similarity of microbial assembly [4] , [5] , also known as the distance–decay relationship or the taxa–area relationship (TAR) [6] . Application of the TAR has demonstrated that the species richness of eukaryotic macroorganisms increases with the sampling area [7] . This significant rate of diversity turnover has generally been explained by a dynamic equilibrium between extinction and immigration (“area” hypothesis, mediated by dispersal) and/or by the increase of habitat diversity with increasing area (“habitat heterogeneity” hypothesis, mediated by environmental selection) [7] . In microorganisms, phylogeographic studies have revealed that the genetic similarity within particular populations decreases with distance, which suggests a significant influence of dispersal limitation, leading to strong endemism [3] , and contradicts the hypothesis of microbial cosmopolitanism [8] . At the community level, biogeographical studies have indicated that diversity turnover is influenced both by geographical distance [9] and environmental heterogeneity (as classified by soil, vegetation and climatic characteristics) [10] , [11] . However, few in-depth studies have been carried out on the TAR of soil microorganisms, especially for soil bacteria, leading to a lack of concepts concerning the diversification processes. TAR was first reported for plants in 1921 by Arrhenius [12] as a power-law relationship: where S A is the number of taxa recorded in an area A , S 0 the initial number of taxa in the smallest sampling area and z is the rate at which new taxa are sampled as the sampling area is increased. TAR was extended to microorganisms less than a decade ago [3] , [9] , [13] by focusing on community similarity between sites: where z is the turnover rate as in equation (1), χ d and χ D are the operational taxonomic unit (OTU bin ) similarities between sites located d meters and D meters apart from each other ( d 2 and D 2 would correspond to the area of the sampled locations), respectively. Nowadays, TAR is commonly used in this form in most microbial biogeographical studies [3] , [9] , [14] , [15] , [16] to assess microbial diversification and its potential relative dependency on “dispersal” and “habitat heterogeneity” (including habitat diversity and landscape configuration) [4] . Nevertheless, the TAR is still highly debated, particularly regarding its form, underlying hypotheses and factors affecting the relationship [17] , [18] , [19] . Rosindell et al. [19] highlighted that the TAR follows a power-law relationship under the hypothesis of infinite community size and for a steady z . As the soil microbial community is very large and diverse [20] , the relationship for these organisms exhibits power-law behaviour because the average abundance per microbial taxonomic unit is large according to Harte et al. [21] On the other hand, the constant z hypothesis across spatial scales, which assumes self-similarity as a probability rule [13] , [18] for the spatial distribution of taxa abundance, may not hold for soil microbes [15] , [21] , [22] . Therefore, z may be considered constant only at a given scale of investigation, not across spatial scales [21] , and such spatial variations must be specified for microbial communities. Now, it is crucial to investigate whether spatial variations of soil bacterial communities observed on a wide scale comply with the Baas Becking postulate [1] involving solely environmental selection as related to habitat-related environmental heterogeneity, or if other ecological processes could be involved in these patterns (for example, dispersal in the context of Neutral Theory). In this context, at least two objectives might be reached, (i) determine the extent to which soil bacterial diversity increases with sampling area by applying TAR from local to wide scales [6] , [23] , and (ii) evaluate the link between biodiversity turnover, environmental heterogeneity and dispersal by confronting community and habitat diversity turnover rates. In this study, we attained these objectives by conducting a wide-scale investigation on a national soil survey: the French Soil Quality Monitoring Network (‘Réseau de Mesures de la Qualité des Sols’, RMQS) that covers the huge environmental diversity of whole France (2,085 sites analysed) [24] . Variations in microbial community between soils were assessed by bacterial Automated Ribosomal RNA Intergenic Spacer Analysis (ARISA) directly on soil DNA [25] . The TAR was then applied to ARISA data by considering the slope ( z bacteria ) together with the initial similarity [5] ( χ 16 ) at the grain size of the study (16 km) and the average similarity as proposed by Morlon et al. [4] to complete the analysis of community spatial variations. In parallel, soil habitat, namely the “description of a physical place, at a particular scale of space and time, where an organism either actually or potentially lives” [26] , was characterized by including pedoclimatic, geomorphologic and land-use data. The TAR concept was then transposed to habitat, assuming that its similarity would decrease with increasing distance (habitat–area relationship (HAR)). For TAR and HAR, the dependence of the slopes and average similarities on spatial scales was evaluated on the scale of France, after which the study of ecological processes was focused on a circular neighbourhood 280 km in diameter. The slopes of the TAR and HAR, as well as the initial similarities and average similarities at this spatial scale, were then confronted and highlighted that dispersal limitation and environmental heterogeneity were not mutually exclusive to determine the bacterial diversity turnover. Soil-sampling network The French Soil Quality Monitoring Network represents 2,085 analysed sites, 2,172,570 pairwise comparisons with distances ranging from 16 km to ca. 1,100 km and covers more than 550,000 km 2 . 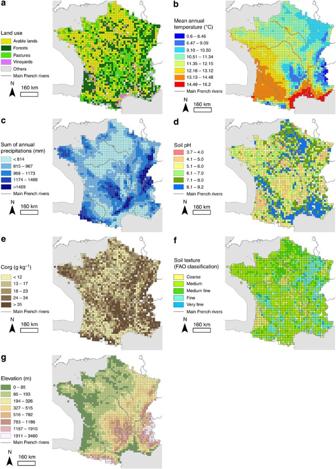Figure 1: Environmental variability across France. (a) Map of land-uses according to the Corine land cover classification; (b,c) maps of climatic conditions: mean annual temperature and sum of annual precipitations, respectively; (d–f) Maps of soil physico-chemical characteristics: pH, organic carbon content and soil texture according to the Food and Agriculture Organization (FAO) classification; (g) map of elevation (m). Through this network, the enormous environmental heterogeneity of France was examined from a huge number of combinations of soil physico-chemical characteristics, geomorphologic characteristics, land uses and climatic conditions ( Table 1 and Fig. 1 ). Table 1 Summary statistics of habitat variables. Full size table Figure 1: Environmental variability across France. ( a ) Map of land-uses according to the Corine land cover classification; ( b , c ) maps of climatic conditions: mean annual temperature and sum of annual precipitations, respectively; ( d – f ) Maps of soil physico-chemical characteristics: pH, organic carbon content and soil texture according to the Food and Agriculture Organization (FAO) classification; ( g ) map of elevation (m). Full size image The range of spatial structures for soil bacterial communities and soil habitat characteristics was estimated by computing experimental variograms for each axis of the principle component analysis (PCA) analyses of bacterial community data and habitat data. 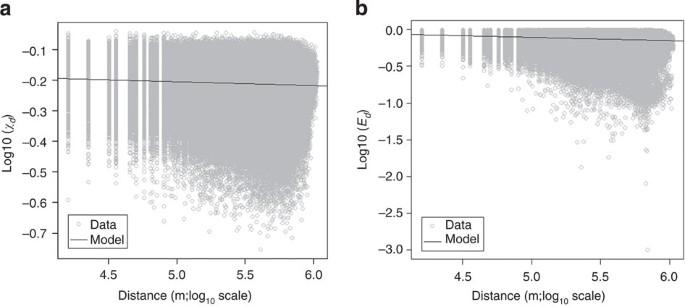Figure 2: TAR and HAR relationships at the scale of France. (a) TAR, (b) HAR, grey circles: logarithm of genetic and habitat similarity values for each paired comparison of sites confronted with the logarithm of between-sites geographical distance (m); black line: weighted linear regression model for the distance–decay relationships. (a) Significant model (P<0.001): log10(genetic similarity)=−0.0117*log10(geographical distance) −0.1464. (b) Significant model (P<0.001): log10(habitat similarity)=−0.0454*log10(geographical distance)+0.1174. The results are presented in Table 2 . The nugget effects were large for bacterial communities (nugget:sill ratio of 0.57 to 0.85) and smaller for soil habitat (nugget:sill ratio of 0.21 to 0.68). The effective variations for the different axes, both for habitat and soil bacterial community, ranged from 150 to 470 km and highlighted large spatial structures. The size of the spatial structures explaining the most the inertia of bacteria and habitat variations (PCA axis 1 in Table 2 ) ranged from 250 to 320 km. Table 2 Fitted parameters of the variograms of bacterial genetic structure and soil habitat. Full size table Distance decay of bacterial community and habitat The TAR measures the spatial turnover of community richness and allows the rate of community composition turnover (commonly referred to as z ) to be calculated. According to Green et al. [9] , z can be equivalently calculated from the increase of community richness with sampled area or from the decay of similarity in the community composition with increasing distance between sampling sites. Here the bacterial community composition of the soil samples was characterized by ARISA and the samples were sorted into OTUs. Bacterial community similarity on the scale of France decreased significantly with geographical distance, indicating that the TAR was significant and demonstrating a spatially structured distribution of soil bacteria over a distance ranging from 16 to 1,100 km ( Fig. 2a ). At this scale, the estimated z bacteria was 0.006 (±7 × 10 −4 , P <0.001). Figure 2: TAR and HAR relationships at the scale of France. ( a ) TAR, ( b ) HAR, grey circles: logarithm of genetic and habitat similarity values for each paired comparison of sites confronted with the logarithm of between-sites geographical distance (m); black line: weighted linear regression model for the distance–decay relationships. ( a ) Significant model ( P <0.001): log 10 (genetic similarity)=−0.0117*log 10 (geographical distance) −0.1464. ( b ) Significant model ( P <0.001): log 10 (habitat similarity)=−0.0454*log 10 (geographical distance)+0.1174. Full size image The turnover rate of habitat ( z habitat ) was determined by transposing the TAR to habitat, assuming that the HAR was a power-law relationship ( Fig. 2b ). Similarly, a significant HAR was also found on the scale of France with an estimated z habitat of 0.023 (±1 × 10 −5 , P <0.001). Influence of spatial scale on TAR and HAR As the parameters (initial similarity and turnover rate) of the TAR, and therefore those of HAR by transposition, might be affected by the spatial scale considered, the regression parameters of the TAR and HAR were compared for different spatial scales (0–70, 70–140, 140–280, 280–560 and 560–1120, km, Fig. 3 ). The z bacteria ranged from 0.003 to 0.010, depending on the scale. The z bacteria was not significantly different at the smallest (0–70 and 70–140 km) and the largest (560–1120, km) scales, but was significantly higher than at the intermediate scales (140–280 and 280–560 km). Conversely, the z habitat presented higher values than the z bacteria (from 0.018 to 0.055) and was positively correlated with spatial scale. Interestingly, z habitat increased moderately and regularly up to the 280–560 km scale, but increased very drastically at scale larger than 580 km. 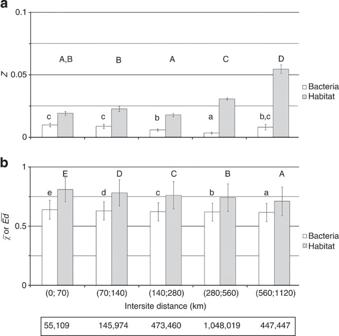Figure 3: Scale effects on TAR and HAR parameters. Variations ofzbacteriaandzhabitat(a), and of the average similarity of bacterial community () or habitat () (b) at different spatial scales. Error bars correspond to 95% intervals for regression parameters (z) and to s.d. for average similarity of bacterial community or habitat. The result of the statistical comparisons ofzor average similarities between spatial scales is indicated through capital letters for habitat and through lower case letters for bacteria. The box at the bottom of the figure indicates the number of pairwise comparisons per spatial scale. Figure 3: Scale effects on TAR and HAR parameters. Variations of z bacteria and z habitat ( a ), and of the average similarity of bacterial community ( ) or habitat ( ) ( b ) at different spatial scales. Error bars correspond to 95% intervals for regression parameters ( z ) and to s.d. for average similarity of bacterial community or habitat. The result of the statistical comparisons of z or average similarities between spatial scales is indicated through capital letters for habitat and through lower case letters for bacteria. The box at the bottom of the figure indicates the number of pairwise comparisons per spatial scale. Full size image The average similarities of bacterial communities and habitat ranged from 0.62 and 0.64 to 0.71 and 0.81, respectively. The ranges of variations were small, even if significant differences were observed between every spatial scale with a decreasing trend from small to large scales. The initial similarities of bacterial community ( χ 16 ) or habitat ( E d16 ) were defined at the grain size of the study (16 km) and could not be calculated over multiple spatial scales. Nevertheless, this metric was compared with the average similarity at different scales. Here, χ 16 and E d16 were 0.65 and 0.84, respectively, representing higher values than the average similarities calculated at different scales. Relationship between initial or average similarities Here the objective was to determine if bacterial similarity was determined by the similarity of habitat at a local spatial scale (16 km) and at the patch scale, that is, if similar habitats house similar bacterial communities. The confrontation of initial similarities ( χ 16 and E d16 , Fig. 4a ) exhibited a relationship modelled with a linear regression type II model. The associated permutation test highlighted the significance of this relationship (1,000 permutations, r 2 =0.123, P <0.001). In this relationship, χ 16 decreased with increasing E d16 , but the range of variations of χ 16 and E d16 remained small. 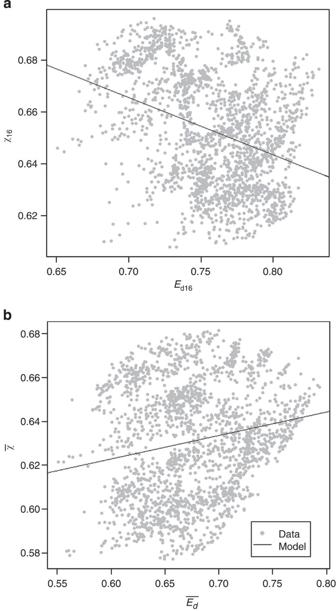Figure 4: Relationship between bacterial communities and habitat similarities. (a) Initial similarities at 16 km; and (b) mean similarity of habitat and bacterial community estimated for each RMQS site considering every site within a circular neighbourhood with a 280 km in diameter. Black line: best significant model fitted to the data (P<0.001, 1,000 permutations): (a) log10(χ16)=−0.2210* log10(?d16)+0.8204, (b)=0.1071 *+0.5586. Figure 4: Relationship between bacterial communities and habitat similarities. ( a ) Initial similarities at 16 km; and ( b ) mean similarity of habitat and bacterial community estimated for each RMQS site considering every site within a circular neighbourhood with a 280 km in diameter. Black line: best significant model fitted to the data ( P <0.001, 1,000 permutations): ( a ) log 10 ( χ 16 )=−0.2210* log 10 (? d16 )+0.8204, ( b ) =0.1071 * +0.5586. Full size image The average similarity of bacterial community structure was significantly correlated to the average habitat similarity ( r 2 =0.036, P <0.05, 1,000 permutations Fig. 4b ), but the range of variations of and remained small. In addition, χ 16 and , and E d16 and were also correlated ( r =0.982 and 0.806, respectively). TAR–HAR relationship The slopes of the TAR and HAR were confronted to evaluate if the turnover rate of soil bacterial community was determined by the turnover rate of soil habitat. To achieve this goal, the statistical confrontation of z bacteria and z habitat was performed by systematically defining TAR and HAR in a neighbourhood corresponding to a circular sliding window of 280 km diameter, centred on each of the 2,085 RMQS sites. The window size was deduced from the size of spatial structures of bacteria and habitat identified by the experimental variograms on the scale of France ( Table 2 ) [27] . The range of variations in z bacteria and z habitat could thus be determined and showed that z bacteria ranged from −0.003 to +0.021 (mean=0.008, median=0.009), whereas z habitat ranged from −0.002 to 0.131. For z bacteria , the negative turnover rates (<1% of total estimates) were observed in some regions where distant sites were more similar to those in the centre, than to intermediate sites. Although in 62% of the regions defined by the sliding windows, the TAR ranged from 0.002 to 0.01 and was close to that observed for France as a whole, in 36% of the regions, the TAR was significantly higher and ranged from 0.01 to 0.02. In other respects, the value of z habitat calculated for France (0.023) was lower than the mean (0.040) or median (0.035) obtained for the 2,085 regions. In some regions (<1%), z habitat was negative because distant sites showed greater similarity to those in the centre than to intermediate sites. Statistical confrontation of the 2,085 z bacteria and z habitat estimates revealed a linear relationship ( Fig. 5 ). The significance of the relationship was tested through a linear regression type II model [28] , as both estimated turnover rates were associated with errors. A permutation test (random association of z habitat and z bacteria values, 1,000 permutations) [29] showed that the model and the regression parameters were highly significant ( r 2 =0.667, P <0.001 and Fig. 5 ). 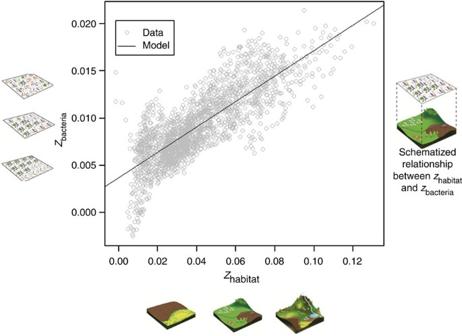Figure 5: Relating turnover rates of soil bacterial community structure and habitat. Grey circles represent the turnover rates calculated for each RMQS site considering every site within a distance of 140 km in a circular window. The black line represents the linear model type II fitted to the data:zbacteria=0.1350 *zhabitat+0.0036, (r2=0.65,P<0.001). Representation of diversity and spatial fragmentation of soil bacterial community assemblage and of habitats are schematized by the y axis and under the x axis, respectively. Figure 5: Relating turnover rates of soil bacterial community structure and habitat. Grey circles represent the turnover rates calculated for each RMQS site considering every site within a distance of 140 km in a circular window. The black line represents the linear model type II fitted to the data: z bacteria =0.1350 * z habitat +0.0036, ( r 2 =0.65, P <0.001). Representation of diversity and spatial fragmentation of soil bacterial community assemblage and of habitats are schematized by the y axis and under the x axis, respectively. Full size image Influence of landscape configuration Habitat turnover rate and initial similarity are determined by habitat diversity and its spatial configuration (that is, landscape configuration). In the previous section, the permutation test demonstrated that habitat diversity significantly influenced the relationship between habitat and bacterial community turnover and initial similarities. Therefore, in this section the objective was to evaluate the importance of landscape configuration on these relationships. To achieve this goal, a permutation test was performed in which the spatial organization of habitat was reconfigured without modifying the bacterial community variability, habitat variability or the selection pressure of habitat on the bacterial community (pairs of habitat and bacterial community composition data unmodified). The modification of landscape configuration significantly altered the correlation ( Fig. 6a ) between z bacteria and z habitat , and changed the sign of the correlation between χ 16 and E d16 in the random case. This might be related to the range of variations of χ 16 , which was smaller than that of E d16 . Similarly, the intercepts of the relationships β z and β χ were significantly reduced by landscape reconfiguration: 0.004 versus 0 and 0.820 versus 0.558, respectively ( Fig. 6c ). The slope of the relationship between the initial similarities ( α χ ) was also affected by landscape reconfiguration (−0.221 versus 0.108 in the random case Fig. 6f ), but this was not the case for the slope α Z that harboured very similar values for the observed and the random cases (0.1350 and 0.1231, respectively, Fig. 6e ). 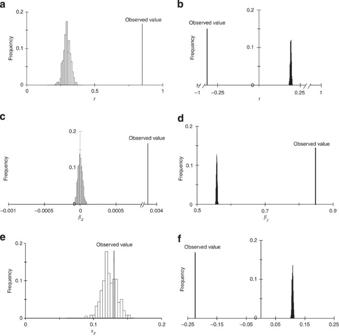Figure 6: Effect of landscape on microbial and habitat turnover rates or initial similarities. (a) Distribution of the correlation coefficient (r) of the relationship between turnover rates; (b) distribution of the correlation coefficient (r) of the relationship between initial similarities; (c) distribution of the intercept (βz) of the relationship between turnover rates; (d) distribution of the intercept (βχ) of the relationship between initial similarities; (e) distribution of the slope (αz) of the relationship between turnover rates; (f) distribution of the slope (αχ) of the relationship between initial similarities. Each distribution is based on 500 permutations in each sliding window. Figure 6: Effect of landscape on microbial and habitat turnover rates or initial similarities. ( a ) Distribution of the correlation coefficient ( r ) of the relationship between turnover rates; ( b ) distribution of the correlation coefficient ( r ) of the relationship between initial similarities; ( c ) distribution of the intercept ( β z ) of the relationship between turnover rates; ( d ) distribution of the intercept ( β χ ) of the relationship between initial similarities; ( e ) distribution of the slope ( α z ) of the relationship between turnover rates; ( f ) distribution of the slope ( α χ ) of the relationship between initial similarities. Each distribution is based on 500 permutations in each sliding window. Full size image In this study, a significant turnover of soil bacterial diversity was demonstrated on a broad scale. This is an important and relevant finding, as several aspects of bacterial physiology and ecology (ubiquity, horizontal gene transfer, high ability to colonize extreme environments, redundancy of ecological attributes) [20] would be expected to prevent a significant TAR for these organisms. Significant TAR have already been reported for indigenous bacteria from various ecosystems, such as water-filled tree holes [30] or salt marshes [14] , which suggests that TAR is a universal relationship for all living organisms and all environments. The estimated z bacteria was 0.006 (±7 × 10 −4 , P <0.001), that is, within the lower range of turnover rates for microbes (0.002< z <0.26), as compiled by Woodcock et al. [31] This is in agreement with the general trend observed for microbes, the values usually being well below than those of the macroorganisms ( z macroorganisms ≥0.1) [14] , even if a higher z bacteria (0.26) has been reported for small, discrete and highly heterogeneous ecosystems [30] known as hosting insular communities with a high community turnover [32] . The significant but low turnover observed on a wide scale in our study might partly be ascribed to the high average abundance per taxonomic unit, which induces low turnover rates [21] , and to technical limitations, particularly the low taxonomic resolution of DNA fingerprinting. Indeed, DNA fingerprints correspond to dominant bands, each including multiple species. This results in an aggregation of species composition variations within the bands and may contribute to the low turnover rate observed [4] . In addition, DNA fingerprinting precludes consideration of the accumulation of new minor species with increasing distance, which may represent a large proportion of the total soil microbial species richness [33] and determine the slope of TAR [14] , [31] . The low z bacteria might also be related to the grain size of our sampling design (16 km × 16 km: 256 km 2 ), which did not consider scales less than landscape, and smoothed significant local variations in soil microbial community composition that might potentially affect TAR [34] . In parallel, soil habitat was characterized by a multivariate analysis including pedoclimatic, geomorphologic and land-use data, and the HAR was calculated by transposing the TAR concept. On the scale of France, z habitat was 0.023 (±1 × 10 −5 , P <0.001). This value can only be considered in relation to z bacteria , as no other means of comparison is available in the literature. The z habitat was higher than the z bacteria , which might be related to the lower average abundance per habitat than per bacterial OTU bin . As described in previous studies, TAR is sensitive to the spatial scale of investigation [21] . The sampling design applied in our study allowed us to test this hypothesis on both TAR and HAR, and to consider multiple spatial scales (distance range between site: [0; 70], [70–140], [140; 280], [280; 560] and [560; 1100] km). The significant effect of spatial scale on the average similarities of soil bacterial community and habitat and on the turnover rates was demonstrated. The average similarities decreased significantly with increasing spatial scale and were always lower than the corresponding initial similarity (0.65 and 0.84 for χ 16 and E d16 , respectively). This is in agreement with the hypothesis that neighbouring sites are more similar than distant sites [2] , [15] . The significant decrease of z bacteria with increasing spatial scales might be explained by the higher average abundance per OTU with increasing scales [21] , [22] . Similarly, the significant increase of z habitat with spatial scale might result from decreasing average abundance per habitat, as the number of observations per habitat increases equally or even more slowly than habitat richness. Altogether, the significant variations of z bacteria and z habitat according to scale might reflect variations in the relative importance of diversification processes [4] . Morlon et al. [4] demonstrated the relevance of distance–decay relationships for testing spatial ecology theories. We therefore compared three metrics relating bacterial community and habitat, namely turnover rates, initial and average similarities, to identify the processes involved in the spatial distribution of soil bacterial communities. These comparisons were performed by computing and compiling data from the 2,085 circular neighbourhoods (280 km in diameter as determined from experimental variograms, see Table 2 ). At this spatial scale, the main processes to consider were (i) environmental heterogeneity leading to adaptation of populations to a particular habitat, the larger areas exhibiting a higher renewal of habitat variation [2] , [30] , that is, the “environmental selection hypothesis”, and (ii) “dispersal limitations” resulting from the balance between species extinction and colonization, which is significantly influenced by the size of the sampling area. If dispersal is infinite, community composition is fully determined by environmental selection, bearing out the postulate of Baas Becking [1] : “Everything is everywhere, but, the environment selects”. Under this postulate, the turnover rate of the soil bacterial community would be entirely proportional to the turnover of the soil environment and would, on average, be zero in completely homogeneous soil environments ( z habitat =0). Otherwise, if the dispersal of soil bacteria is limited, significant turnover rates of bacterial community would be observed in homogeneous habitats according to the Neutral Theory [19] , [35] . Under infinite dispersal, the same interpretation would hold for the relationships between the initial or average similarities of soil bacterial community and habitat, which should be positive and reach the maximum in fully homogeneous habitat. Here the average habitat similarity and average bacterial community similarity were significantly and positively correlated at the scale of the circular neighbourhoods, which was in agreement with the environmental selection hypothesis [2] , [16] , [36] . Nevertheless, the initial similarities of habitat and soil bacterial community were weakly but negatively correlated, suggesting that variations in community composition occur at small scales, even in homogeneous habitats. The significant linear regression between z habitat and z bacteria demonstrated a positive relationship between soil bacterial community turnover and habitat turnover on a regional scale ( Fig. 5 ), thereby supporting the environmental selection hypothesis for soil microorganisms [3] , [7] . It is interesting to note that z bacteria values may attain those reported for larger organisms ( ca. 0.02), even in large areas of contiguous habitats, suggesting that communities of both bacteria and macroorganisms are structured by analogous processes [31] . Recent microbial biogeography studies have revealed that the main environmental filters shaping spatial microbial diversity distribution are soil physico-chemical characteristics, land use and plant cover, whereas climatic and geomorphologic filters are less important [9] , [11] , [15] , [37] . Similar filters were also reported to explain soil bacterial community distribution in contrasted ecological regions at the scale of France [27] , [34] . Nevertheless, the estimated z bacteria in the case of a homogeneous habitat ( z habitat =0) was not equal to 0, suggesting that bacterial communities might have a limited dispersion despite the huge amounts of bacteria (>10 15 cells per year) transported through the atmosphere between continents [38] . This conclusion for the soil bacterial community as a whole is in agreement with phylogeographic studies focusing on particular soil bacterial groups [15] , [16] , [39] and with studies showing a distance effect on soil bacterial community structure [2] . We then determined the relative dependency of bacterial community turnover on dispersal limitation by testing the effect of habitat spatial configuration on the relationships between z bacteria and z habitat , and between the initial similarities ( χ 16 and E d16 ) without modifying the environmental selection process, that is, the pairs of soil habitat characteristics and associated bacterial community composition data. By shuffling habitat spatial configuration, we altered the relationships between turnover rates and between initial similarities of bacterial community and habitat, respectively ( Fig. 6 ). The versatility of the correlation (in terms of sign and significance) between the initial similarities confirmed the difficulty of drawing conclusions at the grain size of this study. On the other hand, the relationship between turnover rates was significantly altered for the correlation and intercept, but not for the slope. This supported the hypothesis that the slope of the relationship between turnover rates is determined by the selection pressure of the soil habitat on the indigenous bacterial community. It also suggested that the intercept of the relationship (bacterial diversity turnover rate in homogeneous habitats) is related to dispersal limitations mediated by the spatial configuration of the habitat. This statement would be in favour to the role of population aggregation in determining the turnover rate of bacterial diversity [4] . Our study negates the hypothesis that the soil microbial community is a “black box” with no spatial structure and exhibiting a homogeneous distribution from local to large scales. As observed in macroorganisms, spatial patterns in soil bacterial communities are also significantly governed by environmental heterogeneity and dispersal, and the two processes are not mutually exclusive [2] , [7] . Moreover, the environmental filters impacting the turnover of soil microbial diversity as a whole need to be deciphered and ranked to better understand the sustainability of the soil ecosystem services provided by the corresponding biodiversity. This represents a major challenge in microbial ecology, but should provide the knowledge required for sustainable soil management and implementation of the corresponding protection policies on a wide scale [40] . Soil-sampling strategy The soil samples were provided by the platform GenoSol ( http://www.dijon.inra.fr/plateforme_genosol ) from the soil storage facility of the RMQS (French Monitoring Network for Soil Quality), which is a soil-sampling network based on a 16 km × 16 km systematic grid covering the whole of France [41] . Each of the 2,195 monitoring sites has been precisely geopositioned, and the soil profile, site environment, climatic factors, vegetation and land use have been accurately described. In the centre of each 16 km × 16 km square, 25 individual core samples were taken from the topsoil (0–30 cm) within a 20 m × 20 m area, using an unaligned sampling design. The core samples were then bulked to obtain a composite sample for each site. The soil samples were gently air-dried, sieved to 2 mm and stored at −40 °C before DNA analysis. Physical and chemical analyses (listed in Table 1 and Fig. 1 ) are available for 2,131 soils and were performed by the Soil Analysis Laboratory of INRA (Arras, France, http://www.lille.inra.fr/las ). Available climatic data were monthly rain, Potential EvapoTranspiration and temperature at each node of a 12 km × 12 km grid, averaged for the 1992–2004 period. These climatic data were obtained by interpolating observational data using the SAFRAN model [42] . The RMQS site-specific data were linked to the climatic data by finding the closest node from the 12 km × 12 km climatic grid for each RMQS site. Land cover was recorded according to the CORINE Land Cover classification at level 1 ( http://www.ifen.fr ), which consists of a rough descriptive classification of land use into five classes: arable lands, forests, pastures, vineyards and other land uses. All these data were available for 2,085 soils in the INRA InfoSol DONESOL database ( http://www.gissol.fr/programme/rmqs/RMQS_manuel_31032006.pdf ; Table 1 and Fig. 1 ). Characterization of habitat Soil habitat was characterized for each site by its coordinates in a Hill and Smith multivariate analysis [43] using the dudi.hillsmith function in the ade4 package [44] in R, which allows mixing quantitative (geomorphological data: altitude, slope and orientation; climatic data: mean annual temperature, annual rainfall and annual potential evapotranspiration; soil physico-chemical data: clay, silt and sand contents, pH water , organic C content, total N content, CaCO 3 content and C:N ratio) and qualitative variables (land use, five classes; Table 1 and Fig. 1 ). Quantitative variables were centred and scaled, and the qualitative variables were converted into binary variables. All the quantitative variables had a weight of 1 in the analysis and the binary variables had a weight equal to 1/ n , n being the number of classes observed in the qualitative variables they were derived from. According to the decrease of inertia per axis, five axes representing 63.9% of the variance in the environmental data were retained to characterize the habitat of each study site. The coordinates of the sites in the Hill and Smith multivariate analysis were used in the following and referred to as habitat characteristics. Molecular characterization of bacterial community structure DNA was extracted from 2,085 soils from the RMQS grid, using a single procedure optimized by Ranjard et al. [25] , which is reliable and robust for the routine analyses of several hundreds of different soils. Soil bacterial community structure was genotyped directly from soil DNA extracts using a bacterial ARISA, fingerprinting approach optimized for medium throughput in the GenoSol platform. Within the ARISA method, the bacterial intergenic spacers were amplified with the primer set: S-D-Bact-1522-b-S-20/ L-D-Bact-132-a-A-18, with 50 ng of DNA as template, the PCR conditions being described by Ranjard et al. [25] The S-D-Bact-1522-b-S-20 primer was labelled at its 5′ end with the IRD800 dye fluorochrome (MWG SA Biotech, Ebersberg, Deutschland) to allow detection of the PCR fragments by the LiCor DNA sequencer system (ScienceTec, Les Ulis, France). PCR fragments were resolved on 3.7% polyacrylamide gels run under denaturing conditions for 15 h at 3,000 V/60 W on a LiCor DNA sequencer (ScienceTec). The data were analyzed using the 1D-Scan software (ScienceTec). This software converts fluorescence data into electrophoregrams where the peaks represent the PCR fragments. The height of the peaks was calculated in conjunction with the median filter option and the Gaussian integration in 1D-Scan, and represented the relative proportions of fragments in the total products. Lengths (in base pairs) were calculated using a size standard with bands ranging from 200 to 1,206 bp. Data obtained from the 1D-Scan software (Sciencetec) were converted into a table summarizing band presence (that is, peaks) and intensity (that is, height or area of peak) using the PrepRISA program [25] . As described in a previous study, 100 peaks, 2 bp resolution and Gaussian peak area were used to provide a robust analysis of bacterial communities [25] . The resulting bacterial-ARISA data matrix (bacterial communities as rows and bands as columns), takes into account the presence/absence and relative intensity of bands. Bacterial community and habitat experimental variograms We used the classical geostatistics approach [45] to characterize the spatial process of bacterial genetic structure and soil habitat. Exponential variograms have been fitted using weighted least squares on the different experimental variograms computed for each axis of the PCAs performed on genetic and environmental data. In this method, the weights of each lag are the experimental variogram of the lag divided by the number of observation pairs within a bin centred on the lag. To characterize the spatial process, we have calculated first the nugget:sill ratio, which represents the non-explanatory part of the spatial model. Second, we retained also the effective range, which is the distance data that the semivariance value achieves 95% of its maximum. TAR and HAR computing The turnover rate of bacterial community composition ( z bacteria ) was determined by converting molecular fingerprint data into presence/absence data and computing between-sites similarity using the dsvdis function (Sørensen index) of the labdsv package [46] in the R software [47] . Then, z bacteria was estimated from the slope of the decay relationship between similarity and distance according to the formula: where χ d is the observed Sørensen’s similarity between two soil samples (number of common OTUs divided by the average number of OTUs in the two samples), which are d meters apart from each other, b is the intercept of the linear relationship and z is the turnover rate of the community composition (referred to as z bacteria ). Regression parameters (−2 z ) and b were estimated by weighted linear regression using the ordinary least squares method. The weight of each similarity value corresponded to the number of data in the respective distance class. This approach was applied to avoid bias related to large distance classes, including few but very dissimilar sites. The significance threshold was set at α =0.05. The turnover rate of habitat ( z habitat ) was determined by transposing the TAR to habitat, assuming that the HAR was a power-law relationship. For this purpose, habitat characteristics were used to compute between sites similarity ( E d ) as follows: with Euc d the Euclidean distance (dist function, R software) between two sites that are d meters apart from each other, and Euc max is the maximum Euclidean distance in the distance matrix; 0.001 was added to account for zero similarity between sites [29] . Then, z habitat was estimated from the slope of the decay relationship between habitat similarity and distance according to equation (3). Regression parameters were calculated by adopting the same methodology used to calculate the parameters for the TAR. Average and initial similarities The average similarity of soil habitat ( ) or of bacterial community composition ( ) was determined as the mean of the similarity matrix computed for soil habitat or bacterial community as described above. The initial similarities of soil habitat ( E d 0 ) or of bacterial community composition ( χ 0 ) were computed as the mean similarity between sites for a distance between sites of 16 km. Relating habitat and bacterial similarities or turnovers To evaluate these relationships, a neighbourhood statistics approach was used allowing computation of z bacteria , z habitat , E d16 , χ 16 , and for each site in the RMQS on a circular neighbourhood 280 km in diameter. For that purpose, the same methods as those presented in the sections devoted to computing the TAR, the HAR, the average and the initial similarities of soil habitat and bacterial community composition were applied. The size and shape of the neighbourhood was in agreement with previous spatial analyses of habitat and genetic data that demonstrated significant spatial structures [27] when the radius was at least 140 km ( Table 2 ). As all the parameters are estimated with errors, the relationships were best modelled by a type II linear regression model (ordinary least squares method). This was done using the ‘lmodel2’ function of the ‘lmodel2’ package [28] in the R software. A permutation test (1,000 permutations) was used to test the significance of the relationship and its parameters [28] . The slope and the intercept were referred as follows: α Z , β Z , α χ , β χ , , for the relationship between z bacteria and z habitat , χ 16 and E d16 , and ; respectively. Influence of landscape configuration To evaluate the influence of landscape on the relationship between habitat and bacterial community turnover or between initial similarities, a permutation test (500 permutations) was performed. In this test, the neighbourhood statistics approach described above was used, but the geographic coordinates of the sites in the neighbourhood region (280 km diameter) were shuffled without modifying the pairs of soil habitat characteristics and bacterial community composition data. This allowed creating randomly configured regions in which bacterial community variability (average similarity and variance), habitat variability (average similarity and variance) and selection pressure of habitat on bacterial community were kept unchanged (pairs of habitat and bacterial community composition data unmodified). As a consequence, only turnover rates and initial similarities were affected, but not the average similarities. Then, the relationships between turnover rates or between initial similarities were computed for each permutation. As a result, the distributions of the Pearson’s correlation coefficient and of the regression parameters ( α Z , β Z , α χ , β χ ) were considered for each relationship. Then, the probability of observed value were derived from these distributions and confronted to the 5% significance threshold. How to cite this article: Ranjard, L. et al. Turnover of soil bacterial diversity driven by wide-scale environmental heterogeneity. Nat. Commun. 4:1434 doi: 10.1038/ncomms2431 (2013).